Cell wall precursors are required to organize the chlamydial division septum Members of the Chlamydiales order are major bacterial pathogens that divide at mid-cell, without a sequence homologue of the FtsZ cytokinetic tubulin and without a classical peptidoglycan cell wall. Moreover, the spatiotemporal mechanisms directing constriction in Chlamydia are not known. Here we show that the MreB actin homologue and its conserved regulator RodZ localize to the division furrow in Waddlia chondrophila, a member of the Chlamydiales order implicated in human miscarriage. RodZ is recruited to the septal site earlier than MreB and in a manner that depends on biosynthesis of the peptidoglycan precursor lipid II by the MurA enzyme. By contrast, crosslinking of lipid II peptides by the Pbp3 transpeptidase disperses RodZ from the septum. Altogether, these findings provide a cytological framework for understanding chlamydial cytokinesis driven by septal cell wall synthesis. Fundamental to proliferation of all cells, the molecular basis of cell division in Chlamydiales is still largely uncharted territory. While several proteins that are essential for division in other bacteria are not encoded in the chlamydial genomes, functional studies on chlamydial cell division are hampered by their poor genetic tractability and their obligate intracellular lifestyle. The Chlamydiae are composed of the members of the Chlamydiaceae family and of several other family-level lineages coined ‘ Chlamydia -related bacteria’. Chlamydiaceae include major human pathogens: C. trachomatis causes urogenital infections and trachoma; C. pneumoniae and C. psittaci cause pneumonia [1] . Waddlia chondrophila , another member of the Chlamydiales order, is implicated in abortion in bovines [2] and in miscarriage in humans [3] , [4] , [5] . Like other Chlamydiae , W. chondrophila is a strict intracellular bacterium that exhibits two developmental states: infectious non-dividing elementary bodies (EBs) and non-infectious dividing reticulate bodies (RBs) [6] , [7] , [8] . When EBs enter cells, they reside in a vacuole called inclusion. Next, they differentiate into RBs, decondensing their genome and initiating transcription and replication. Finally, RBs redifferentiate into EBs that are expelled by exocytosis or cell lysis [8] . W. chondrophila represents an ideal model for cytological studies on Chlamydiae . W. chondrophila can infect and proliferate in a range of cells, including amoebae, human macrophages, Vero cells, pneumocytes, endometrial cells and fish cell lines [9] , [10] , [11] , [12] , presumably because of the larger metabolic capacity encoded in its genome versus that of Chlamydiaceae [13] . Moreover, Waddlia cells are bigger than those of Chlamydiaceae and thus better suited for protein localization studies underlying chlamydial cell division. Unlike Chlamydiaceae , W. chondrophila is resistant to many β-lactam antibiotics [10] that target the bacterial cell wall (peptidoglycan). Peptidoglycan (PG) is a polymer of glycan strands assembled from N-acetyl-glucosamine and N-acetyl-muramic acid through β-(1,4)-glycosidic bonds and stabilized through peptide bridges containing D -amino acids. While it protects cells from lysis in hypo-osmotic conditions and endows cells with their characteristic shape, it also plays an important role in cell division as PG synthesis at the division septum (septal PG) can direct the invagination of the cytoplasmic membrane [14] . Recently, PG has been biochemically detected in Chlamydiae , and circumstantial evidence suggests that PG-like material resides at the chlamydial division septum [15] , [16] . Moreover, functional homologues of PG biosynthesis enzymes are encoded in chlamydial genomes [17] , [18] , [19] , [20] , [21] . Septal PG is likely produced in low amounts, in a modified form and/or only transiently during constriction, explaining why it is difficult to detect by conventional biochemical techniques. Antibodies raised against mycobacterial cell wall skeleton detect a septal non-proteinaceous antigen, likely a derivative of PG [22] , in dividing Chlamydiae. The apparent absence of coding sequences for enzymes that typically catalyse the polymerization of the glycan strands, suggests that Chlamydiae might, alternatively, polymerize a modified PG structure composed exclusively of crosslinked peptide bridges without a glycan component [18] . Nevertheless, penicillin-binding protein (Pbp) homologues that are responsible for the trans-peptidation of neighboring penta-peptide bridges are encoded in Chlamydiae , and penicillin inhibits division and induces the formation of large abnormal RBs, called aberrant bodies [23] . Aberrant bodies may result from continued DNA replication without division, the counterpart of filamentous cells arising when division of rod-shaped bacteria is inhibited by penicillin. Importantly, aberrant bodies are involved in the persistence of chlamydial infections and are also induced by iron or nutrient starvation or by IFN-gamma treatment [23] , [24] , [25] , [26] . When stress is relieved, aberrant bodies divide into RBs, which can further differentiate into EBs [27] , indicating that viability is maintained to a certain degree when division is inhibited. In most bacteria, septal PG synthesis is organized by the FtsZ division protein, a tubulin homologue that polymerizes into a membrane-associated contractile ring at the future division site and that recruits cell division proteins including the PG biosynthetic machine. The FtsZ (Z-) ring can also invaginate the cytoplasmic membrane, at least in vitro [28] . Remarkably, Chlamydiae divide by binary fission [7] , [8] , [9] , [22] in the absence of a FtsZ sequence homologue [13] , [29] . Furthermore, the C. trachomatis genome has only three annotated cell division genes: ftsI (encoding Pbp3), ftsK and ftsW , whereas the W. chondrophila genome encodes sequence homologues of ftsI , ftsK , ftsL , ftsQ and ftsW . Although Chlamydiae lack FtsZ, they do encode homologues of the MreB actin and its regulator RodZ, known to be involved in cell shape control by regulating PG synthesis in rod-shaped bacteria [30] . Importantly, a functional and cytological relationship between RodZ and the cytokinetic Z-ring has been described [31] , [32] , [33] , [34] . In the absence of a FtsZ-cytoskeleton, Chlamydiae might rely on MreB and/or RodZ to organize division. Since MreB can polymerize in vitro , it is a good candidate to act as a cytoskeletal element that could organize chlamydial division [35] . Several MreB interactors were described; FtsK directly interacts with the C. trachomatis MreB (in a bacterial two-hybrid (BACTH) assay [36] ), MreC interacts with a MreB homologue in Bacillus subtilis [37] and with RodZ, which was shown to anchor MreB to the membrane in E. coli [38] and which is uncharacterized in Chlamydiales [39] . Moreover, E. coli MurG, a component of the PG biosynthesis pathway, also interacts with MreB [40] and Chlamydia pneumoniae MreB interacts with MurG and MraY by BACTH assay and with MurF in an in vitro cosedimentation assay [35] . However, the spatial relationship between these factors and the chlamydial division septum remains unexplored. Here, we show that MreB and RodZ are localized to the division septum in W. chondrophila RBs. Interestingly, septal localization of RodZ precedes that of MreB and is dependent on the function of MurA, a critical enzyme of the PG biosynthesis pathway, which can be inhibited by the phosphonic antibiotic phosphomycin. RodZ is enriched at mid-cell upon penicillin treatment, indicating that RodZ is an early component of the septum, which then recruits other components of the division machinery, possibly MreB, which may provide the driving force for the final stages of division before Pbp3 disperses RodZ. Taken together, our data highlight the important role of PG derivatives or precursors in organizing chlamydial division septum. Primary structure and function of chlamydial MreB Bioinformatics revealed that chlamydial MreBs exhibit 51.8–59.3% identity with the orthologues of Escherichia coli , Thermotoga maritima and Caulobacter crescentus . Moreover, as many as 92.3% of the known active site residues [41] were conserved in all six species investigated, whereas only 33.8% of the complete MreB sequences were conserved ( P <0.001, supplementary Fig. 1A ), and important features that were shown to be required for MreB interaction with the bacterial membrane, an amphipathic N-terminal helix and a hydrophobic hairpin, are also conserved among all Chlamydiales [42] ( Supplementary Fig. 1A ). Consistent with the notion that chlamydial MreB has MreB-like functional properties, we observed that overexpression of W. chondrophila MreB (MreB Wc ) in wild-type C. crescentus induced a ‘lemon-shape’, a loss of crescent shape and swelling of the cell similar to that caused by depletion of MreB from Caulobacter (MreB Cc ) ( Supplementary Fig. 1B ) [33] . While MreB Wc could not substitute for MreB Cc , the trans-dominance suggests that MreB Wc can interfere with MreB Cc . As the MreB Wc -induced loss of crescent shape and swelling resembles those of C. crescentus cells following treatment with the MreB inhibitors, A22 and MP265 (ref. 43 ), we explored the effect of A22 and MP265 on W. chondrophila and C. pneumoniae . As A22 and MP265 might disturb the host cell cytoskeleton because of the homology between MreB and actin, we tested the effect of actin and tubulin inhibitors cytochalasin D and nocodazole on Waddlia growth. These compounds are toxic for the host cell ( Supplementary Fig. 1C ) but do not inhibit proliferation of W. chondrophila ( Supplementary Fig. 1D,E ). While A22 or MP265 have minor toxic side-effects on Vero and Hep-2 host cell ( Supplementary Fig. 1C ), division and replication of W. chondrophila in Vero cells and of C. pneumoniae in Hep-2 cells were impaired after administering either drug at 2 h post-infection (p.i.) ( Fig. 1a and Supplementary Fig. 1F ). Consistent with our findings, inhibitors of MreB disturb infection by Chlamydia trachomatis [36] . We cannot exclude that this growth defect is partially due to toxicity of the drugs towards the host cell, but more than 80% of the host cells were still viable at a dose that inhibited the bacterial growth by 99%. Moreover, we observed the presence of aberrant bodies in cells treated with MP265 for both W. chondrophila and C. pneumoniae ( Fig , arrows and Supplementary Fig. 2A ). Addition of the drugs at 12 and 24 h p.i. caused a rapid block of W. chondrophila proliferation ( Supplementary Fig. 2B–E ), indicating that the drugs likely do not affect the bacteria at a specific step of bacterial infection such as entry, differentiation or exit of the bacteria but likely act on bacterial division. Moreover, mitochondrial recruitment 8 h p.i. was not prevented by these drugs as shown by Mitotracker staining ( Supplementary Fig. 2F ). Interestingly, when the drugs were added 2 h p.i. and removed 24 h p.i., Waddlia replicated again by budding from aberrant bodies ( Supplementary Fig. 2I , arrows), showing that A22 and MP265 are bacteriostatic ( Supplementary Fig. 2G,H ). 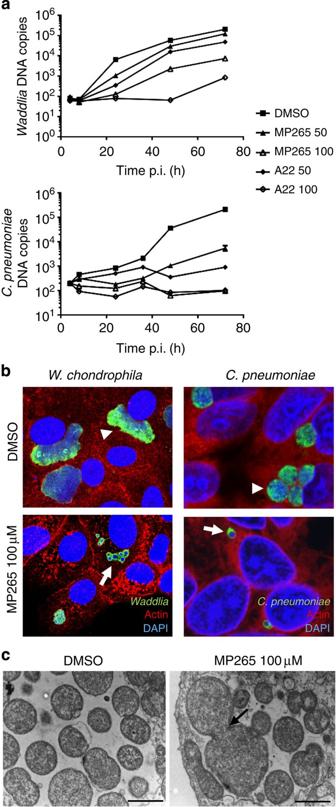Figure 1: MreB inhibition blocks chlamydial infection and induces aberrant bodies formation. (a) DNA replication rate is lower in presence of the MreB inhibitors. Vero cells (resp. Hep-2 cells) were harvested at different time points after infection withW. chondrophila(resp.C. pneumoniae) with or without treatment with A22 or MP265 (50 or 100 μM), DNA was extracted andW. chondrophila(resp.C. pneumoniae) DNA was quantified by qPCR. (Error bars represent the s.d. of three independent experiments). (b) Treatment ofW. chondrophilawith MreB inhibitors induces the formation of aberrant bodies. Infected Vero cells (resp. Hep-2 cells) were fixed and stained with anti-Waddliaantibodies (resp. anti-chlamydial LPS antibodies), anti-Actin antibodies and DAPI. Confocal microscopy was performed 48 h p.i. in absence or presence of MP265. Normal inclusions filled with dividing RBs are pointed by arrowheads, whereas enlarged non-dividing aberrant bodies are pointed by arrows. (c) Aberrant bodies ofW. chondrophilaobserved by electron microscopy. Infected Vero cells were treated with MP265 2 h p.i. Cells were harvested 24 h p.i., fixed and prepared for EM as described. The arrow points the presence of an aborted invagination at the mid-cell (Scale bar, 1 μm). Figure 1: MreB inhibition blocks chlamydial infection and induces aberrant bodies formation. ( a ) DNA replication rate is lower in presence of the MreB inhibitors. Vero cells (resp. Hep-2 cells) were harvested at different time points after infection with W. chondrophila (resp. C. pneumoniae ) with or without treatment with A22 or MP265 (50 or 100 μM), DNA was extracted and W. chondrophila (resp. C. pneumoniae ) DNA was quantified by qPCR. (Error bars represent the s.d. of three independent experiments). ( b ) Treatment of W. chondrophila with MreB inhibitors induces the formation of aberrant bodies. Infected Vero cells (resp. Hep-2 cells) were fixed and stained with anti- Waddlia antibodies (resp. anti-chlamydial LPS antibodies), anti-Actin antibodies and DAPI. Confocal microscopy was performed 48 h p.i. in absence or presence of MP265. Normal inclusions filled with dividing RBs are pointed by arrowheads, whereas enlarged non-dividing aberrant bodies are pointed by arrows. ( c ) Aberrant bodies of W. chondrophila observed by electron microscopy. Infected Vero cells were treated with MP265 2 h p.i. Cells were harvested 24 h p.i., fixed and prepared for EM as described. The arrow points the presence of an aborted invagination at the mid-cell (Scale bar, 1 μm). Full size image Localization of MreB and RodZ to the division septum To determine the subcellular localization of MreB and its potential regulators/interactors FtsK, FtsQ, MreC and RodZ, we raised antibodies against recombinant His 6 -tagged variants purified from E. coli . Of these candidates, only RodZ and MreB showed an expression and localization consistent with a cytokinetic role ( Supplementary Fig. 3A ). Both antisera recognize a single protein of the expected size by immunoblotting ( Supplementary Fig. 3B ), and biochemical fractionation experiments by ultracentrifugation followed by immunoblotting showed the protein to reside in the predicted subcellular compartments. MreB is present both in the membrane (insoluble) and cytoplasmic (soluble) fraction, consistent with the known partitioning properties of monomeric and polymeric MreB, respectively. By contrast, RodZ partitioned exclusively to the membrane fraction, consistent with the C-terminal membrane spanning fragment predicted for residues 110–128 of RodZ ( Supplementary Fig. 3C ). Quantitative reverse-transcriptase PCR (qRT–PCR) measurements revealed a peak of mreB and rodZ transcripts between 8 and 24 h p.i. but otherwise constant expression ( Fig. 2a ). Indeed, immunoblotting ( Fig. 2b ) and immunofluorescence microscopy ( Fig. 2c ) showed that MreB and RodZ are present throughout the developmental cycle, although RodZ abundance in EBs (discernible from RBs by virtue of their condensed nucleoid) appeared reduced by immunofluorescence ( Fig. 2c , arrows). 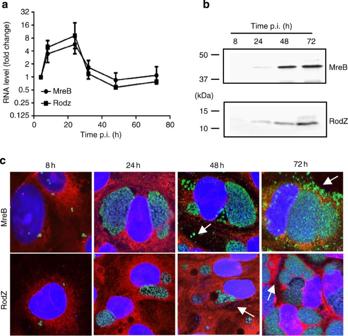Figure 2: MreB and RodZ are synchronously expressed, but RodZ does not accumulate in EBs. (a) RNA expression of MreB and RodZ are synchronous. Vero cells were infected withW. chondrophila, and samples were taken at the indicated time points. RNA was extracted, cDNA was synthesized and quantified by qPCR as described (Error bars represent the s.d. of three independent experiments). (b) Antibodies against MreB and RodZ are specific. Similar samples as forawere taken and proteins were extracted. Proteins were then detected by western blot with antibodies raised against purified MreB or RodZ. (c) MreB protein is detectable in both EBs and RBs but RodZ only in RBs during the developmental cycle. Vero cells infected with W. chondrophilawere fixed at the given time points and labelled with an anti-MreB antibody (green), concanavalin A (red) and DAPI (blue) and observed by confocal microscopy. Arrows point to extracellular EBs, which can be recognized thank to their condensed DNA. Figure 2: MreB and RodZ are synchronously expressed, but RodZ does not accumulate in EBs. ( a ) RNA expression of MreB and RodZ are synchronous. Vero cells were infected with W. chondrophila , and samples were taken at the indicated time points. RNA was extracted, cDNA was synthesized and quantified by qPCR as described (Error bars represent the s.d. of three independent experiments). ( b ) Antibodies against MreB and RodZ are specific. Similar samples as for a were taken and proteins were extracted. Proteins were then detected by western blot with antibodies raised against purified MreB or RodZ. ( c ) MreB protein is detectable in both EBs and RBs but RodZ only in RBs during the developmental cycle. Vero cells infected with W . chondrophila were fixed at the given time points and labelled with an anti-MreB antibody (green), concanavalin A (red) and DAPI (blue) and observed by confocal microscopy. Arrows point to extracellular EBs, which can be recognized thank to their condensed DNA. Full size image To determine the localization of these proteins during division, we observed dividing bacteria 28 h p.i., a time at which RBs are dividing but no redifferentiation to EBs is visible. We classified the dividing bacteria into early, medium or late dividing cells depending on the morphology of the septum (open septum for early, closed septal band for medium and a single septal focus for late, Fig. 3a ). We observed MreB to be enriched at the division septum only at medium and late division stages ( Fig. 3b,d ). To exclude that this fluorescence signal is due to MreB in juxtaposed neighbouring cytoplasmic membranes of the two daughter cells, we quantified the fluorescence signal along dividing cells. We observed an increase in the MreB fluorescence signal at the septum compared with the fluorescence signal obtained with the polyclonal polyspecific antibodies directed against all immunogenic Waddlia proteins (‘total’ anti- Waddlia , Fig. 3d lines 1–3). Moreover, quantification of signals along the division septum shows a different distribution of MreB compared with that of total anti- Waddlia signal ( Fig. 3d , lines 4–6). Taken together, the septal signal stemming from the anti-MreB antibody exceeds that from the other antibodies including the total anti- Waddlia , anti-FtsQ, anti-FtsK and anti-MreC antibodies. 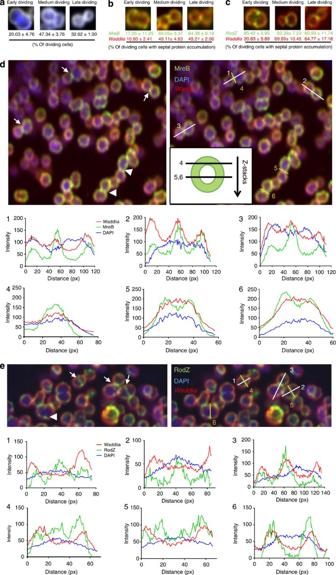Figure 3: RodZ accumulates at the division septum earlier during division than MreB. (a) DividingW. chondrophilaare classified into three groups: early, medium and late division. Vero cells were infected withW. chondrophila, fixed 28 h post-infection and labelled with a total anti-Waddliaantibody and DAPI. Dividing bacteria were then observed and quantified by confocal microscopy (N=200). (b) MreB localizes at the division septum only during medium and late dividing stages. Infected cells were treated as inabut labelled with anti-MreB antibodies (green) and total anti-Waddliaantibodies (red) and quantified by confocal microscopy (N=100). (c) RodZ localizes at the division septum early during division. Infected cells were treated as inabut labelled with anti-RodZ antibodies (green) and total anti-Waddliaantibodies (red) and quantified by confocal microscopy (N=100). (d) Observation of dividingW. chondrophilaby confocal microscopy shows different MreB-containing structures: line (arrows) and distinct punctuae (arrowheads). Quantification of the fluorescence along the described axes (1–6) was performed using Image J software and shown in the corresponding graphs. Longitudinal quantification showed an enrichment of MreB at the dividing plane compared with the totalWaddliasignal (1–3). Transversal quantification along the division septum showed one or two peaks of MreB fluorescence, consistent with a Z-ring structure (4–6). (e) Quantification of the enrichment of RodZ at the division site. The same procedure as indwas performed with an antibody against RodZ. Longitudinal quantification (1–3) showed an enrichment of RodZ at the division septum. Transversal quantification (4–6) shows two peaks characteristic of a Z-ring structure. Figure 3: RodZ accumulates at the division septum earlier during division than MreB. ( a ) Dividing W. chondrophila are classified into three groups: early, medium and late division. Vero cells were infected with W. chondrophila , fixed 28 h post-infection and labelled with a total anti- Waddlia antibody and DAPI. Dividing bacteria were then observed and quantified by confocal microscopy ( N =200). ( b ) MreB localizes at the division septum only during medium and late dividing stages. Infected cells were treated as in a but labelled with anti-MreB antibodies (green) and total anti- Waddlia antibodies (red) and quantified by confocal microscopy ( N =100). ( c ) RodZ localizes at the division septum early during division. Infected cells were treated as in a but labelled with anti-RodZ antibodies (green) and total anti- Waddlia antibodies (red) and quantified by confocal microscopy ( N =100). ( d ) Observation of dividing W. chondrophila by confocal microscopy shows different MreB-containing structures: line (arrows) and distinct punctuae (arrowheads). Quantification of the fluorescence along the described axes (1–6) was performed using Image J software and shown in the corresponding graphs. Longitudinal quantification showed an enrichment of MreB at the dividing plane compared with the total Waddlia signal (1–3). Transversal quantification along the division septum showed one or two peaks of MreB fluorescence, consistent with a Z-ring structure (4–6). ( e ) Quantification of the enrichment of RodZ at the division site. The same procedure as in d was performed with an antibody against RodZ. Longitudinal quantification (1–3) showed an enrichment of RodZ at the division septum. Transversal quantification (4–6) shows two peaks characteristic of a Z-ring structure. Full size image Strikingly, while MreB is a late recruit to the division septum, RodZ localizes to the septum early during division (in more than 80% of early dividing cells, Fig. 3c ). Quantification of the fluorescence signal from the anti-RodZ antibody along the longitudinal ( Fig. 3e , lines 1–3) and transversal axes ( Fig. 3e , lines 4–6) in dividing cells is consistent with a specific septal localization, rather than a diffuse localization in the membrane. Importantly, the total anti- Waddlia antibody did not yield septal staining at this time ( Fig. 3e , lines 1 and 2). Later, in deeply constricted cells, both RodZ and MreB show a similar focal enrichment at the septum ( Fig. 3d lines 1–3 and Fig. 3e line 3). These findings provide strong evidence that RodZ is an early septal protein, while MreB is recruited to the septum only in deeply constricted cells. Septal localization of RodZ is prevented by phosphomycin To explore whether the cell wall biosynthesis enzymes modulate the septal recruitment of RodZ or MreB in Chlamydiae , we first determined the effects of phosphomycin and penicillin (two PG biosynthesis inhibitors) on chlamydial division. Phosphomycin targets MurA, an UDP-N-acetylglucosamine enolpyruvyl transferase, while penicillin inhibits Pbp2 and Pbp3, two peptidoglycan-synthesizing transpeptidase homologues. C. trachomatis MurA is active in vitro and can substitute for E. coli MurA, but is resistant to phosphomycin [44] . In E. coli MurA, resistance to phosphomycin is conferred by a single Cys115 to Asp mutation [45] , a mutation that is present in the MurA orthologues of the Chlamydiacea e, but not in W. chondrophila MurA ( Supplementary Fig. 4 ), suggesting that W. chondrophila should be sensitive to phosphomycin. W. chondrophila encodes a beta-lactamase that should confer some resistance to penicillin derivatives [13] . Nevertheless, we found that W. chondrophila cells are sensitive to each drug at concentrations higher than 100 μg ml −1 ( Fig. 4a,b ), preventing cytokinesis and inducing the formation of aberrant bodies ( Fig. 4c ). In comparison, there was no effect of phosphomycin on growth and morphology of C. pneumoniae ( Fig. 4d,f ), while penicillin had a strong effect on C. pneumoniae growth at much lower concentrations (5–10 μg ml −1 , Fig. 4e ). The penicillin derivatives mecillinam (targeting specifically Pbp2) and piperacillin (acting on Pbp3) partially block both W. chondrophila and C. pneumoniae infections ( Supplementary Fig. 5A–G ). This is consistent with a requirement of both Pbps in chlamydial division, as proposed for C. trachomatis [36] . Taken together, these results confirm that the PG biosynthesis pathway is essential for proper growth of the Chlamydiales . 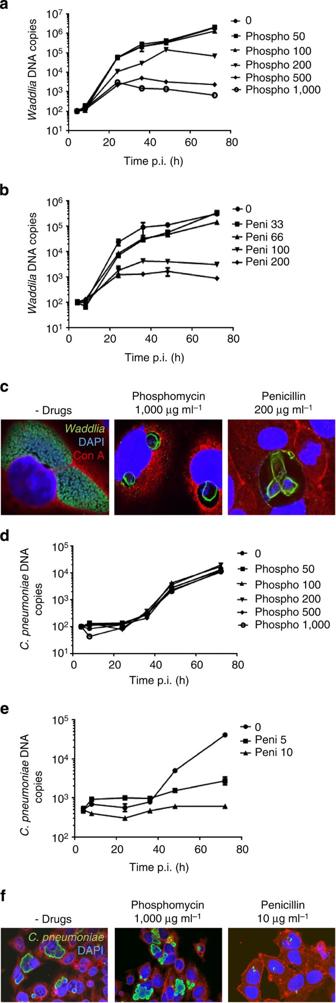Figure 4: Phosphomycin and penicillin block growth ofW. chondrophilaand induce aberrant bodies formation, but only penicillin has an effect onC. pneumoniae. (a)WaddliaDNA replication rate is lower in the presence of phosphomycin. Vero cells infected withW. chondrophilawere harvested at different time points post infection with or without treatment with phosphomycin (50–1,000 μg ml−1), DNA was extracted andWaddliaDNA was quantified by qPCR. (Error bars represent the s.d. of three independent experiments). (b)WaddliaDNA replication rate is lower in the presence of penicillin.Waddlia-infected Vero cells were treated with 0–200 μg ml−1of penicillin 2 h post infection, DNA was extracted at the given time points andWaddliaDNA was quantified by qPCR. (c) High concentrations of phosphomycin and penicillin induce the formation of aberrant bodies inW. chondrophila. Infected Vero cells were fixed and stained with anti-Waddliaantibodies (green), concanavalin A (red) and DAPI (blue). Confocal microscopy was performed 48 h p.i. in absence or presence of the indicated drugs. (d)C. pneumoniaeis resistant to phosphomycin. Hep-2 cells were infected withC. pneumoniae. Phosphomycin (50–1,000 μg ml−1) was added 2 h post-infection. DNA was extracted at the indicated time points andC. pneumoniaeDNA was quantified by qPCR. (e)C. pneumoniaeis sensitive to penicillin. Hep-2 cells were infected withC. pneumoniaeand 5-10 μg ml−1penicillin was added 2 h post-infection. DNA was extracted at the indicated time points andC. pneumoniaeDNA was quantified by qPCR. (f)C. pneumoniaemorphology is not affected by high concentrations of phosphomycin, but aberrant bodies are formed after treatment with penicillin. Hep-2 cells were treated as ind,e. After 24 h, they were fixed and labelled with DAPI, anti-chlamydial LPS antibody (green) and concanavalin A (red) and observed by confocal microscopy. Figure 4: Phosphomycin and penicillin block growth of W. chondrophila and induce aberrant bodies formation, but only penicillin has an effect on C. pneumoniae . ( a ) Waddlia DNA replication rate is lower in the presence of phosphomycin. Vero cells infected with W. chondrophila were harvested at different time points post infection with or without treatment with phosphomycin (50–1,000 μg ml −1 ), DNA was extracted and Waddlia DNA was quantified by qPCR. (Error bars represent the s.d. of three independent experiments). ( b ) Waddlia DNA replication rate is lower in the presence of penicillin. Waddlia -infected Vero cells were treated with 0–200 μg ml −1 of penicillin 2 h post infection, DNA was extracted at the given time points and Waddlia DNA was quantified by qPCR. ( c ) High concentrations of phosphomycin and penicillin induce the formation of aberrant bodies in W. chondrophila . Infected Vero cells were fixed and stained with anti- Waddlia antibodies (green), concanavalin A (red) and DAPI (blue). Confocal microscopy was performed 48 h p.i. in absence or presence of the indicated drugs. ( d ) C. pneumoniae is resistant to phosphomycin. Hep-2 cells were infected with C. pneumoniae . Phosphomycin (50–1,000 μg ml −1 ) was added 2 h post-infection. DNA was extracted at the indicated time points and C. pneumoniae DNA was quantified by qPCR. ( e ) C. pneumoniae is sensitive to penicillin. Hep-2 cells were infected with C. pneumoniae and 5-10 μg ml −1 penicillin was added 2 h post-infection. DNA was extracted at the indicated time points and C. pneumoniae DNA was quantified by qPCR. ( f ) C. pneumoniae morphology is not affected by high concentrations of phosphomycin, but aberrant bodies are formed after treatment with penicillin. Hep-2 cells were treated as in d , e . After 24 h, they were fixed and labelled with DAPI, anti-chlamydial LPS antibody (green) and concanavalin A (red) and observed by confocal microscopy. Full size image Next, we determined the effect of inhibiting PG biosynthesis on septal localization of MreB and RodZ. To this end, we treated infected cells 2 h p.i. with phosphomycin or penicillin and immunostained cells for RodZ and MreB in the resulting aberrant bodies at 24 h p.i. Phosphomycin, but not penicillin, caused a loss of septal localization of RodZ ( Fig. 5 and Supplementary Fig. 5H–K ). After penicillin treatment, more than 30% of aberrant bodies were partially constricted and showed a strong septal localization of RodZ ( Fig. 5 , arrows). Septal RodZ and cell constriction were rarely seen after phosphomycin treatment (in 12.3% of counted bacteria, Fig. 5 ). Interestingly, piperacillin but not mecillinam had a similar effect on RodZ localization as penicillin ( Fig. 5b and Supplementary Fig. 5L,M ). This indicates that Pbp3, rather than Pbp2, plays a role in the recruitment of the Waddlia division machinery and that its inhibition causes an accumulation of septal RodZ. Moreover, MurA acts upstream of Pbps to localize RodZ to the septum because addition of both phosphomycin and penicillin together results in a similar localization defect of RodZ as phosphomycin alone ( Fig. 5 ). This is consistent with the fact that MurA is also biochemically upstream of Pbps in the PG biosynthetic pathway. Interestingly, addition of MP265 also blocks RodZ accumulation ( Fig. 5 ). Thus, RodZ depends on MreB to reach the septum or to be retained at this site (see discussion). 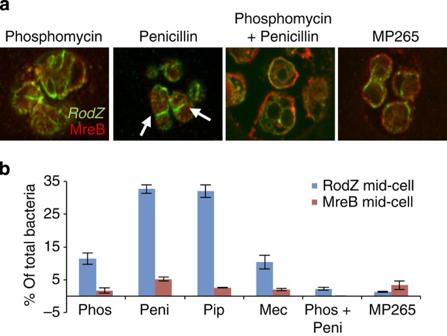Figure 5: Effect of phosphomycin, penicillin and MP265 on the localization of RodZ and MreB. (a) Localization of RodZ and MreB in presence of different drugs. Vero cells infected withW. chondrophilawere treated with the indicated drugs 2 h p.i. (500 μg ml−1phosphomycin, 500 μg ml−1penicillin or 100 μg ml−1MP265). Cells were fixed 24 h p.i., labelled with antibodies against RodZ (green) and MreB (red) and observed by confocal microscopy. Arrows show the accumulation of RodZ at mid-cell. (b) Quantification of the accumulation of RodZ and MreB at the bacterial mid-cell by confocal microscopy after treatment with 500 μg ml−1phosphomycin (Phospho), 500 μg ml−1penicillin (Peni), 500 μg ml−1piperacillin (Pip), 500 μg ml−1mecillinam (Mec) and 100 μg ml−1MP265 (n=100). (Error bars represent the s.d. of three independent experiments). Figure 5: Effect of phosphomycin, penicillin and MP265 on the localization of RodZ and MreB. ( a ) Localization of RodZ and MreB in presence of different drugs. Vero cells infected with W. chondrophila were treated with the indicated drugs 2 h p.i. (500 μg ml −1 phosphomycin, 500 μg ml −1 penicillin or 100 μg ml −1 MP265). Cells were fixed 24 h p.i., labelled with antibodies against RodZ (green) and MreB (red) and observed by confocal microscopy. Arrows show the accumulation of RodZ at mid-cell. ( b ) Quantification of the accumulation of RodZ and MreB at the bacterial mid-cell by confocal microscopy after treatment with 500 μg ml −1 phosphomycin (Phospho), 500 μg ml −1 penicillin (Peni), 500 μg ml −1 piperacillin (Pip), 500 μg ml −1 mecillinam (Mec) and 100 μg ml −1 MP265 ( n =100). (Error bars represent the s.d. of three independent experiments). Full size image While the organization of the chlamydial division septum has remained mysterious in the past, our study makes three major contributions in illuminating the spatiotemporal mechanisms of chlamydial division. First, we unearth RodZ and MreB as the first known septal proteins, with RodZ being an early recruit while MreB follows later. Second, we show that cell wall precursor synthesis and trans-peptidation are required for the septal localization of RodZ and its subsequent dispersion. Finally, we show that cell wall precursor synthesis (lipid II) is required for division in W. chondrophila , suggesting that cell wall promotes constriction. The finding that MreB is involved in the division of Waddlia chondrophila and Chlamydia pneumoniae , two distant members of the Chlamydiales order, is supported by the strong conservation of MreB, by its localization at the periphery of the cell and by its enrichment at the division furrow. A potential role of MreB in the division of C. trachomatis was already proposed by Ouellette and colleagues [36] , based on A22/MP265-treated C. trachomatis cells. We extend these pharmacological results by showing that A22/MP265 also impairs division of W. chondrophila and C. pneumoniae . Importantly, we bolster these findings by showing that MreB localizes to deeply constricted septa. As MreB is not recruited to the division septum early, it does not seem to function as an organizer of early division events as would be expected from a functional homologue of FtsZ. By contrast, we observed an early localization of RodZ to the division septum and an intricate dependence of its localization on the function of PG biosynthesis enzymes in Chlamydiales . Given the ability of RodZ to directly interact with monomeric and filamentous MreB [33] , [34] , [46] , [47] , [48] , we speculate that RodZ could function as the division organizer, tracking or being transported along actin-like filaments of MreB to reach and ultimately mark the future division site. The RodZ protein is usually composed of three conserved domains: a N-terminal essential domain, a transmembrane domain and a dispensable C-terminal domain [39] . The chlamydial RodZ, which exhibits only a low similarity to E. coli RodZ (24–30%, Supplementary Fig. 6A ), has a predicted transmembrane domain but completely lacks the C-terminal domain ( Supplementary Fig. 6B ). The C-terminal part of RodZ is not essential for RodZ localization but is important for its function and stability [39] . Thus, the finding that MreB inhibitors impair RodZ localization to the septum suggests direct interactions between RodZ and MreB; however, indirect explanations are also possible (see below). Recently, it was hypothesized that Chlamydiales synthesize a modified version of PG from Lipid II without glycans [21] . We took advantage of the sensitivity of W. chondrophila to phosphomycin to test whether MurA, a critical enzyme in PG precursor biosynthesis, is required for chlamydial division. Inhibition of MurA with phosphomycin inhibits cytokinesis, resulting in the formation of large, round and unconstricted aberrant bodies, resembling the treatment with the penicillin derivatives that inhibit Pbps. When Pbp3 is inhibited, aberrant bodies with a partial contraction at mid-cell are visible. Finally, when MreB is blocked, partial contraction of aberrant bodies is visible, but RodZ does not accumulate at mid-cell. Thus, MurA, Pbp2 and MreB all seem to be required for proper localization of RodZ at the division septum, while Pbp3 is responsible for a later event that leads to the contraction of the septum and the disassembly of RodZ. This interpretation is strengthened by the result that MurA acts upstream of the Pbps in the W. chondrophila cell wall biosynthesis, because cotreatment with phosphomycin and penicillin causes a phenotype similar to phosphomycin alone. Spatial cues could be provided by enzymes responsible for the synthesis of lipid II, including particularly those that are known to interact with chlamydial MreB such as MurG, MurF and/or MraY [35] , or other proteins that act in an early step of PG biosynthesis [46] . Our result that lipid II plays a key role in the (direct or indirect) organization of the chlamydial division septum is reminiscent of the role of staphylococcal cell wall-associated teichoic acids in organizing division and is in agreement with an unpublished report that Pbp1A and Pbp2X are delocalized from the streptococcal division septum by the lipid II-sequestering antibiotic nisin [47] . Taken together, our results show the importance of cell wall precursors for the organization of the division septum in W. chondrophila . We took advantage of the rapid growth of W. chondrophila , of the bigger size of its cells and of its sensitivity to phosphomycin to perform this study. The resistance of Chlamydiaceae to phosphomycin would not have allowed the investigation of the importance of PG in the division of these bacteria. However, PG precursor biosynthesis is conserved among Chlamydiales ( Supplementary Tables 1 and 2 ), indicating that our results might be representative of a common mechanism among all Chlamydiales . Antibodies, probes and reagents Polyclonal mouse and rabbit antibodies against W. chondrophila were produced in-house as previously described [48] . Antibodies against actin were purchased from Sigma-Aldrich (St Louis, MO). MitoTracker Red CMXRos (M7512) as well as secondary antibodies Alexa Fluor 488 goat anti-rabbit, 488 anti-mouse, 594 anti-rabbit and 594 anti-mouse were all obtained from Molecular Probes (Grand Island, NY). A22, phosphomycin, penicillin, mecillinam and piperacillin were purchased from Sigma-Aldrich. MP265 was synthesized by American Custom Chemicals Corporation (San Diego, CA). Vero cells were treated with 10 μM nocodazole (Sigma-Aldrich) or 10 μM cytochalasin D (Sigma-Aldrich). Primers and probes used in this study are described in supplementary Table 3 . Strains and growth conditions E. coli EC100D (Epicentre Technologies, Madison, WI) and Rosetta (DE3)/pLysS (Novagen, Madison, WI) were grown in Luria Bertani broth (LB). Caulobacter crescentus NA1000 (ref. 49 ) and derivatives were grown at 30 °C in PYE (peptone-yeast extract) or PYE supplemented with either 0.3% xylose (PYEX) or 0.2% glucose (PYEG). W. chondrophila ATCC VR-1470 T was grown using the amoeba Acanthamoeba castellanii ATCC 30010 cultivated in 25 cm 2 cell-culture flasks with 10 ml peptone-yeast extract-glucose medium. The flasks were incubated for 6 days at 28 °C, cell suspension was collected and filtered through a 5-μm-pore filter to retain amoebae and to purify bacteria in the flow-through. C. pneumoniae ATCC VR-1310 was grown using Hep-2 cells cultivated in 24 well-plates (Corning, NY) with 1 ml DMEM containing 10% fetal calf serum (FCS), 1% amino-acid mix, 1% vitamin mix and 2 μg/ml of cycloheximide (Life technologies, Carlsbad, CA). The flasks were incubated for 72 h at 37 °C in presence of 5% CO 2 . Cells were then resuspended and homogenized with glass beads. Cell culture and bacterial infection Vero cells (ATCC CCL-81) were grown in 75 cm 2 flasks with 20 ml DMEM containing 10% fetal calf serum at 37 °C in presence of 5% CO 2 . Hep-2 cells (ATCC CCL23) were grown in 75 cm 2 flasks with 20 ml DMEM containing 10% fetal calf serum, 1% non-essential amino-acid mix, 1% vitamin mix and 2 μg ml −1 of cycloheximide at 37 °C in presence of 5% CO 2 . Overnight cell cultures containing originally 10 5 cells per ml were infected with a 2,000 × dilution of W. chondrophila or a 10 × dilution of C. pneumoniae (MOI of 1-2). The cells were then centrifuged for 15 min ( W. chondrophila ) or 30 min ( C. pneumoniae ) at 1,790 g , incubated 15 min at 37 °C, washed with PBS before addition of fresh media. Immunofluorescence labelling Infected Vero or Hep-2 cells on coverslips were fixed with ice-cold methanol for 5 min at room temperature or with 4% paraformaldehyde for 15 min. Mitotracker staining was performed on living cells before fixation following the manufacturer’s protocol (Molecular Probes). After fixation, cells were washed three times with PBS. Cells were then blocked and permeabilized for at least 1 h with a blocking buffer (PBS, 0.1% saponin, 1% BSA). Coverslips were then incubated with 1:100 dilutions of primary antibodies directed against bacteria or the actin of the host diluted in blocking buffer for 1 h at room temperature. After three washes with PBS containing 0.1% saponin, coverslips were incubated with 1:1,000 dilutions of secondary antibodies in blocking buffer containing DAPI (Molecular Probes). Coverslips were washed three times with PBS containing 0.1% saponin, once with PBS and once with water. Subsequently, they were mounted onto glass slides using Mowiol (Sigma-Aldrich) [48] , [50] . Confocal and fluorescence microscopy Infection rate, inclusions and aberrant bodies were quantified by fluorescence microscopy by counting a minimum of hundred cells in duplicate. Images were taken by confocal microscopy using a Zeiss LSM 510 Meta (Zeiss, Oberkochen, Germany). Images were then treated and quantified using the ImageJ software ( http://www.macbiophotonics.ca ). Quantitative PCR Infection was quantified by real-time PCR. At different time points after infection, infected cells were resuspended by scrapping. Genomic DNA was extracted from 50 μl of cell suspension using the Wizard SV Genomic DNA purification system (Promega, Madison, WI). Elution was processed with 200 μl of water. Quantitative real-time PCR was performed using iTaq supermix with ROX (BioRad, Hercules, CA). To detect W. chondrophila , 200 nM of primers WadF4 and WadR4, 100 nM of probe WadS2 (ref. 51 ) and 5 μl of DNA were used. For C. pneumoniae detection, 550 nM of primers CpnF and CpnR, and 100 nM of probe CpnS were used [52] . Cycling conditions were 3 min at 95 °C followed by 40 cycles of 15 s at 95 °C and 1 min at 60 °C for both PCRs. A stepOne Plus Real-time PCR System (Applied Biosystems, Carlsbad, CA) was used for amplification and detection of the PCR products. RNA extraction, cDNA synthesis and qPCR Five hundred microlitres of infected cell culture was taken at the given time points, mixed with 1 ml of RNA Protect (Qiagen, Venlo, Netherlands), mixed and incubated for 5 min at room temperature. The suspension was then centrifuged for 10 min at 5,000 g , the supernatant was removed and the pellet was frozen at −80 °C. The pellet was then unfrozen, and RNA was extracted using the RNeasy Plus kit (Qiagen). DNA contamination was removed by DNAse digestion, using Ambion DNA-free kit (Life technologies, Grand Island, NY). cDNA was then synthesized by reverse transcription using a Goscript Reverse Transcription System (Promega, Fishburg, WI). qPCR was performed by adding 4 μl of cDNA to 10 μl of iTaq Universal SYBR Green mix (BioRad, Hercules, CA), 4.8 μl of water and 0.6 μl of each specific forward and reverse primers targeting the 16S rRNA gene, mreB or rodZ . Cycling conditions were 3 min at 95 °C followed by 45 cycles of 15 s at 95 °C and 1 min at 60 °C. A stepOne Plus Real-time PCR System (Applied Biosystems, Carlsbad, CA) was used for amplification and detection of the PCR products. Protein extraction, SDS-PAGE, western blot Five-hundred microlitres of infected cell culture were harvested at different time points. Cells were harvested, and proteins were extracted by resuspension in loading buffer (60 mM Tris pH 6.8, 1% SDS, 1% mercaptoethanol, 10% glycerol, 0.02% bromophenol blue). Ten microlitres of the suspension was loaded on a 12.5% polyacrylamide gel. After 45 min migration at 200V, proteins were transferred onto a nitrocellulose membrane by electroblotting at 75 V for 1 h. The membrane was blocked with 5% milk for 2 h and then incubated for at least 2 h with a 1:2,500 dilution of rabbit antibody directed against heat-inactivated W. chondrophila . An incubation of 2 h with a 1:2,500 dilution of a HRP-conjugated goat anti-rabbit antibody was then performed. Detection of HRP was done using 0.03% hydrogen peroxide, 220 μg ml −1 luminol and 32.5 μg ml −1 coumaric acid in 0.1 M Tris pH 8.5. Chemiluminescence was recorded with the ImageQuant LAS 4000 Mini imager (GE healthcare, Waukesha, WI). Images were then treated using ImageJ. Uncropped version of the Western blot is provided in the Supplementary Fig. 3B . Electron microscopy Vero and Hep-2 cells were infected as described above. Infected cells were collected 24 h p.i. and fixed in 2% paraformaldehyde and 0.1% glutaraldehyde for 45 min. Samples were then treated for 1 h at room temperature with 1% osmium tetroxide in PBS and then washed several times in increasing acetone concentrations (50–100%). Samples were resuspended for 1 h in acetone–epon and overnight in epon and finally embedded using an epoxy resin (Fluka). Embedded blocks were then sliced with a LKB 2088 Ultratome microtome, placed on formvar-coated copper grids (Sigma–Aldrich) and stained for 10 min with methanol–uranyl acetate and lead nitrate with sodium citrate in water [48] . The resulting sections were examined with a Philips CM-100 transmission electron microscope. Bioinformatic studies Identity values were obtained using BLASTP version 2.2.25 with an expectation value threshold of 0.1. If necessary, the average identity of multiple High-Scoring segment Pair (HSP) was weighted according to the length of each HSP. Protein sequences were aligned using Tcoffee [53] . The computational analyses were performed at the Vital-IT ( http://www.vital-it.ch ) Center for high-performance computing of the Swiss Institute of Bioinformatics (SIB). Amphipathic helixes prediction was done using the online program Amphipaseek ( http://npsa-pbil.ibcp.fr/ ) [54] . Topology and transmembrane domain prediction was performed using the online program TMHMM Server ( http://www.cbs.dtu.dk/services/TMHMM/ ) Cell viability Viability of the host cells in presence of the different drugs was determined using the Resazurin kit (Sigma-Aldrich). Cells were incubated for 24 h in presence of the drugs. Resazurin was added in an amount equal to 10% of the culture volume. Cells were then incubated at 37 °C for 4 h. Absorbance was then measured using the FLUOstar Omega microplate reader (BMG Labtech, Offenburg, Germany). MreB expression, purification and antibody production mreB Wc was amplified from W. chondrophila ATCC VR-1470 (ref. 13 ) genomic DNA by using primers mreB_Nde and mreB_Eco . The product was digested with NdeI and EcoRI restriction endonucleases (Roche, Basel, Switzerland) and the reaction purified with QIAquick Gel extraction kit (QIAgen, Venlo, The Netherlands). The purified mreB Wc was ligated into the expression vector pMT335 (ref. 55 ) restricted with NdeI and EcoRI. Recombinant plasmids were introduced in E. coli EC100D by electroporation. The construct was verified by sequencing (Fasteris, Geneva, Switzerland). His 6 -SUMO-MreB Wc was expressed in pCWR547 in E. coli Rosetta (DE3)/pLysS and purified under denaturing conditions (in 8 M UREA standard procedures, QIAgen, Hilden, Germany). In brief, cells were inoculated in 1 l of LB and grown at 30 °C until they reached an OD 600 = ∼ 0.4. One millimolar IPTG was added to the culture and then grown at 30 °C for 3 h. Cells were pelleted and resuspended in 25 ml of lysis buffer (10 mM Tris HCl pH8, 0.1 M NaCl, 1 mM β-mercaptoethanol, 5% glycerol, 0.5 mM imidazole, triton 0.02%). Cells were sonicated (Sonifier Cell Disruptor B-30; Branson Sonic Power , Danbury, CT) on ice using 20 bursts of 20 s at output level 5.5. After centrifugation at 6,000 r.p.m. for 20 min at 4 °C, the supernatant was discarded while the pellet was resuspended in buffer B (8 M Urea, 0.1 M NaH 2 PO 4 , 0.1 M Tris-HCl, pH 8.0). The resulting suspension was centrifuged for 20 min at 6,000 r.p.m. at 4 °C. The supernatant was loaded onto a column containing 5 ml of Ni-NTA agarose resin. Column was rinsed with buffer B and buffer C (8 M Urea, 0.1 M NaH 2 PO 4 , 0.1 M Tris-HCl, pH 6.3). His 6 -SUMO-MreB Wc was eluted in buffer E (8 M Urea, 0.1 M NaH 2 PO 4 , 0.1 M Tris-HCl, pH 4.5). The protein was then excised from a 12.5% SDS polyacrylamide gel and used to immunize New Zealand white rabbits (Josman LLC, Napa, CA). RodZ expression, purification and antibody production The ORF corresponding to RodZ (ORF wcw_0755) was amplified by PCR using the primers RodZ_fwd and RodZ_rev and cloned into the pET200 vector (Life technologies) in E. coli . This vector allows the expression of a N-terminal tagged version of the protein under a isopropyl-β- D -thiogalactopyranoside (IPTG) inducible promoter. Protein was expressed with 1 mM IPTG (MP Biomedicals, Santa Ana, CA) during 4 h and purified in presence of 8 M urea. Bacteria were lysed using Fastbreak Lysis buffer (Promega). Lysate was then incubated with MagneHis Ni particles beads and beads were washed with binding/wash buffer (Promega). The purified protein was then eluted using 500 mM imidazole (Sigma-Aldrich) [56] . The purified protein was then used to immunize mice (Eurogentec, Seraing, Belgium). Membrane fractionation Waddlia -infected Vero cells were harvested and resuspended in 500 ml of 10 mM EDTA at pH 9.5 and incubated for 2 h at 37 °C. Membrane and cytosol fractions were separated by ultracentrifugation for 1 h at 100,000 g . The membrane and cytosol fraction were boiled in sample buffer and analysed by western blot. How to cite this article: Jacquier, N. et al. Cell wall precursors are required to organize the chlamydial division septum. Nat. Commun. 5:3578 doi: 10.1038/ncomms4578 (2014).